Making head or tail of cnidarianhoxgene function 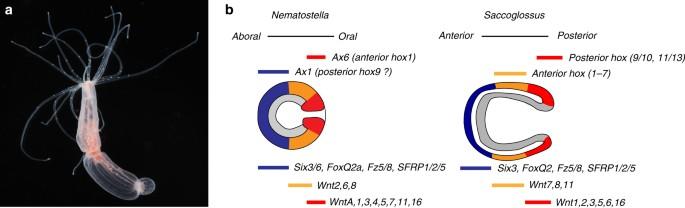Fig. 1 Nematostellaand the evolution of axial patterning systems.aA photograph of an adultNematostella vectensispolyp. A ring of tentacles that are used for capturing prey surrounds the oral opening (oriented to the top). The “oral” opening serves as both mouth and anus and derives directly from the blastopore (to the right inb).bSchematic drawing of gastrula stages ofNematostella vectensisand the hemichordateSaccoglossus kowalevskii, which serves as an example for a bilaterian embryo. The blastopore is oriented to the right. Relative gene expression domains are indicated to illustrate the support for different scenarios in the evolutionary relation of the primary body axis. Note that the gene expression domains are simplified and that some of theNematostellaWnts are expressed in the endoderm. Data forNematostellaare summarized in refs.5,12,13, and forSaccoglossusin ref.15. Photo credit fora: Chiara Sinigaglia Distantly related animals have spectacularly different shapes and body plans, which can render it difficult to understand which of their body parts may have a shared evolutionary origin. Studying the molecular regulation of the development of these body parts during embryogenesis can help identifying commonalities that are not visible by eye. A new study employs this approach to address a fundamental question, the origin of the head-to-tail axis of bilaterians. The results show that two Hox genes—key regulators of the patterning of this axis in bilaterians—have important roles in axial patterning in a sea anemone, which belongs to a group of animals that diverged from the bilaterian lineage more than 600 million years ago. Here, we discuss the implications of these interesting new findings in the light of previous observations on axial patterning in bilaterian and non-bilaterian animals. The body plan of bilaterians (e.g. vertebrates, arthropods and many worm-shaped animals) can be described by a Cartesian coordinate system with three body axes [1] : the anterior–posterior (AP) axis that is oriented parallel to the gut, the dorsal–ventral (DV) axis defining the “back” and “belly” sides and the left–right (LR) axis for laterality. Increasing evidence indicates that the molecular basis of the formation and patterning of these axes is highly conserved within bilaterians, suggesting that at least the AP and DV axes were present already in the last common ancestor of bilaterians. For the AP axis, Wnt/β-Catenin signalling determines the site of gastrulation and endomesoderm formation, and it suppresses anterior and promotes posterior ectodermal development [2] . Interesting and longstanding questions are the relation of the bilaterian body axes to those of pre-bilaterians and the transition from radial to bilateral symmetry in animal evolution [3] , [4] . Here, cnidarians (i.e. jellyfish, hydroids, corals and sea anemones) are of critical importance: they represent the well-established sister group to all bilaterian animals and they exhibit a gastrula-like body plan with a primary radial symmetry [5] (Fig. 1a ). Morphological characters that identify the orientation of the AP axis in most bilaterians (i.e. an anterior brain-like centralization of the nervous system and a through gut with the mouth located anterior to the anus) are not present in cnidarians. A key question is, therefore, which of the molecular vectors (i.e. signalling networks and transcription factors) defining the bilaterian body axes are acting in cnidarian axis formation. Fig. 1 Nematostella and the evolution of axial patterning systems. a A photograph of an adult Nematostella vectensis polyp. A ring of tentacles that are used for capturing prey surrounds the oral opening (oriented to the top). The “oral” opening serves as both mouth and anus and derives directly from the blastopore (to the right in b ). b Schematic drawing of gastrula stages of Nematostella vectensis and the hemichordate Saccoglossus kowalevskii , which serves as an example for a bilaterian embryo. The blastopore is oriented to the right. Relative gene expression domains are indicated to illustrate the support for different scenarios in the evolutionary relation of the primary body axis. Note that the gene expression domains are simplified and that some of the Nematostella Wnts are expressed in the endoderm. Data for Nematostella are summarized in refs. [5] , [12] , [13] , and for Saccoglossus in ref. [15] . Photo credit for a : Chiara Sinigaglia Full size image In an interesting and important recent paper, DuBuc et al. [6] have addressed the role of two Hox genes in axis formation and oral/aboral markers in the sea anemone Nematostella vectensis , which is a major cnidarian model system [5] . Hox transcription factors have a conserved role in the patterning of the bilaterian AP axis [7] . There are three groups of bilaterian Hox genes: anterior, central and posterior ones. They have sharp anterior borders of expression, whereas the posterior limit of their expression is often less clearly defined. The position of the anterior expression border differs for different groups of Hox genes: those of anterior Hox genes are located more anteriorly than those of central and posterior Hox genes. The picture emerging from functional studies (mainly in arthropods and vertebrates) is that Hox genes act from gastrulation stages onwards to provide specific identities to consecutive territories along the AP axis, with the exception of the anterior-most region, which is typically free of Hox gene expression. While Hox genes are essential for the patterning of large parts of the AP axis, they have no role in the initial establishment of the body axis [7] . Cnidarian Hox genes have been identified 26 years ago [8] and reveal a broad spectrum of expression patterns, but only now the first functional analysis of Hox genes during cnidarian embryonic development has been presented by DuBuc et al. [6] . Cnidarians have anterior, but no central, Hox genes and they have genes that have been classified as posterior in some studies and as unresolved non-anterior genes in others [5] , [9] , [10] . DuBuc et al. focus on one anterior ( NvAx6 ) and one putative posterior ( NvAx1 ) Hox gene in Nematostella [6] . In situ hybridization analyses show opposing expression patterns of NvAx1 and NvAx6 . NvAx1 is expressed in blastulae at the presumptive aboral side and Nv Ax6 at the presumptive oral side. In NvAx1 knockdown animals, the expression of aboral-most genes is lost, whereas broader aboral markers ( NvSix3/6 ) and oral markers are not or only slightly affected. Upon knockdown of NvAx6 , the animals fail to complete gastrulation, and the expression of oral markers, including four Wnt genes, is lost. The domain of NvWnt2 (the most aboral cnidarian Wnt gene) is shifted towards the oral pole, but still present. Since knockdown of NvAx1 and NvAx6 results in an expansion of NvAx6 and NvAx1 , respectively, the authors tested by double knockdown whether the expanded expression contributes to the observed phenotypes. After double knockdown, the animals gastrulate, form an endodermal tissue layer and display normal expression of oral genes at gastrula stage (although not at later stages). Unexpectedly, however, the expression of the aboral gene NvSix3/6 is lost in double knockdowns at the gastrula stage, even though single knockdowns show a mild reduction ( NvAx1 ) and expansion ( NvAx6 ), respectively. In overexpression experiments, injection of NvAx1 mRNA suppresses NvAx6 expression, whereas NvAx6 mRNA injection does not suppress NvAx1 . These experiments clearly show that NvAx1 is required for aboral and NvAx6 for oral development in Nematostella and that they mutually inhibit each other’s expression. The relation between Wnt signalling and NvAx6 function remains to be determined, since the earliest analyses of the functional perturbations of the Nematostella Hox genes are performed at the gastrula stage, after the patterning of the oral domain at the blastula stage [11] . Nevertheless, the new data unambiguously show that Hox genes function in the development of the oral–aboral axis in Nematostella . Hox genes and the evolutionary origin of the bilaterian AP axis What does this mean for the evolutionary relation of the oral–aboral axis of cnidarians to the AP axis of bilaterians? The authors suggest that the roles of a Nematostella anterior Hox gene in oral, and a putative posterior Hox gene in aboral development support homology of the cnidarian oral to bilaterian anterior, and aboral to posterior domains. Challenging this hypothesis requires a closer look at the similarity to the role of Hox genes in bilaterians, and, importantly, consideration of existing data on axial patterning in Nematostella and other cnidarians. NvAx1 and NvAx6 appear to function during the blastula stage and they are required for oral-most ( NvAx6 ) and aboral-most ( NvAx1 ) development, while the identity in the domains in between the two poles (based on gene expression, e.g. NvWnt2 ) is unchanged, though displaced towards the oral pole. This is different from the conserved role of bilaterian Hox genes, which act during and after gastrulation, confer a molecular identity to consecutive areas and have no role in anterior-most development. Despite these differences, it is not inconceivable that the function of the Hox system in cnidarians (as described by DuBuc et al. [6] ) and in bilaterians (in AP patterning) had a shared evolutionary origin. The hypothesis devised by DuBuc et al. [6] is, however, contradicted by several publications on the molecular control of axial patterning in Nematostella and other cnidarians. In Nematostella , Wnt genes are expressed exclusively in the oral domain from blastula stages on and β-catenin is nuclearized predominantly in the oral area [4] , [5] , [12] . Wnt signalling is required for endomesoderm development and the genes expressed in the oral domain are most sensitive to reductions of Wnt/β-catenin signalling at the blastula stage [5] , [12] , [13] . These Wnt functions in oral development are strikingly similar to those in posterior development of bilaterians and well conserved in other cnidarians [2] . In contrast, development of the aboral domain requires protection from high levels of Wnt/β-catenin signalling. The transcription factors NvSix3/6 and NvFoxQ2 and the Wnt modulators NvSFRP1 and NvFz5/8 are expressed in the anterior domain of nearly all bilaterians that have been studied and their Nematostella orthologs are expressed in the aboral domain [5] , [13] . The establishment of this domain at blastula stage requires low level Wnt/β-catenin signalling and MAPK activity [13] , [14] . Subsequently, NvSix3/6 and, to a lesser extent, NvFoxQ2a control the further development of the domain, whereas NvFz5/8 prevents the expansion of the aboral domain towards more oral regions [5] , [13] . These data support the hypothesis that with respect to the molecular regulation of axial patterning, the aboral domain of cnidarians is homologous to the anterior domain in bilaterians, and the oral domain to the posterior domain (Fig. 1b ). This would mean that the roles of NvAx1 and NvAx6 in axial patterning evolved independently of those of Hox genes in bilaterians. The remarkable and uncommon early roles of Hox genes in Nematostella identified by DuBuc et al. highlight, however, that the axial patterning systems of cnidarians and bilaterians (and within the two groups) are not simply copies of each other, but rather have undergone substantial modifications during their independent evolution. In future studies, appreciating both conserved and divergent aspects of axial patterning mechanisms will certainly benefit the understanding of their evolution. With respect to Wnt signalling and the Hox genes, it will be interesting to address the mutual effects of manipulating Wnt signalling and NvAx6 at earlier blastula stages, when patterning of the oral–aboral axis commences. Other important questions are the molecular mechanism that localizes Wnt/β-catenin signalling components to the animal domain in Nematostella , but to the vegetal pole in bilaterians [4] , [5] , and the function of other Nematostella Hox genes, whose staggered expression along the secondary body axis resembles bilaterian-type Hox expression more than that of NvAx1 and NvAx6 [4] , [10] . Undoubtedly, the work by DuBuc et al. will serve as an important reference for any new studies on axial patterning in cnidarians, which may ultimately help us in understanding the evolutionary origin of bilaterally symmetric body plans.